Using light transmission to watch hydrogen diffuse Because of its light weight and small size, hydrogen exhibits one of the fastest diffusion rates in solid materials, comparable to the diffusion rate of liquid water molecules at room temperature. The diffusion rate is determined by an intricate combination of quantum effects and dynamic interplay with the displacement of host atoms that is still only partially understood. Here we present direct observations of the spatial and temporal changes in the diffusion-induced concentration profiles in a vanadium single crystal and we show that the results represent the experimental counterpart of the full time and spatial solution of Fick's diffusion equation. We validate the approach by determining the diffusion rate of hydrogen in a single crystal vanadium (001) film, with net diffusion in the [110] direction. Diffusive motion is one of the most intriguing and investigated phenomena in physics. Fick formulated his two laws of diffusion [1] to which Einstein provided a microscopic foundation by considering atoms and molecules undergoing Brownian motion [2] . The interstitial diffusion of hydrogen in metals can be described in an analogous way, in which the motion results from discrete jumps between interstitial sites. The jump- and diffusion-rates are, therefore, intrinsically linked. As a consequence, the diffusion of hydrogen in metals can be inferred from measurements of jump rates in thermodynamic equilibrium, using, for example, nuclear magnetic resonance or quasi-elastic incoherent neutron scattering [3] . Determination of non-equilibrium diffusion can be performed by mechanical relaxation methods, such as the Gorsky effect [3] . Although these techniques have been extremely useful for determining the rate of hydrogen diffusion, they suffer from a severe shortcoming: the results do not provide any information about the evolution of concentration profiles in the samples. This severely limits the possibilities of validating many of the assumptions used when modelling the diffusion of hydrogen in materials. The use of optical techniques to determine position resolved migration of hydrogen was pioneered by den Broeder et al . [4] , utilizing the metal to insulator transition in yttrium hydrides [5] . They could infer the diffusivity of hydrogen by following the frontier of the hydride formation as a function of position and time, by using the large change in the optical transmission resulting from the metal-insulator transition. Later, the same research group developed an approach based on an yttrium coating, whereby the metal insulator transition was used as a marker for the integrated flux of hydrogen in an underlying polycrystalline vanadium film [6] . Both approaches allowed the determination of the speed of the diffusion front, while no information could be obtained about the underlying concentration profiles. Here we present a method that provides time-resolved determination of the diffusion-induced concentration profiles in any metal, that exhibits hydrogen-induced changes of the density of states in the conduction band. The results are compared with the solution of the diffusion equation, and we will show that these provide full information about the development of the hydrogen content in the sample. Concentration conversion and geometrical aspects A schematic illustration of the sample geometry and the instrument is shown in Fig. 1 . The sample is covered with an amorphous aluminum oxide layer, except for a small opening at one end of the sample. The oxide is catalytically inactive and acts as a dissociation and diffusion barrier [7] . At t = t 0 , molecular hydrogen is introduced into the evacuated chamber, which results in a selective dissociation of hydrogen on the catalytically active palladium surface. Atomic hydrogen is thereby introduced at one end of the sample and starts migrating laterally through the vanadium film. Vanadium exhibits a much stronger affinity for hydrogen, as compared with palladium, whereby the concentration in palladium can be safely neglected [3] , [8] . Hydrogen causes changes in the electronic structure, giving rise to changes in the optical transmission, which can be used to determine the concentration [9] , [10] (for further details see the Methods section). The optical transmission is monitored as a function of time using a charge-coupled device, with a lateral resolution of about 20 μm, whereby the concentration of hydrogen as a function of both position and time can be determined. 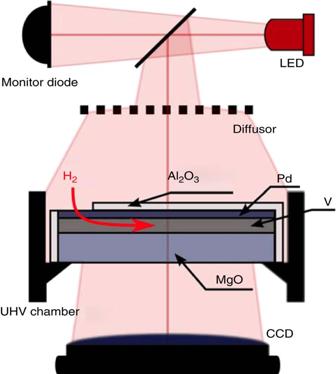Figure 1: Schematic illustration of the experimental approach. Monochromatic light, emitted by a light-emitting diode, shines on a semitransparent mirror, which is used to split the beam allowing simultaneous measurements of the transmission through the sample and the intensity of the source. A diffusor is used to homogenize the illumination, before the entry window of the ultrahigh vacuum chamber. The transmitted light is registered by a CCD camera. The sample is covered with Al2O3to prevent hydrogen from entering and leaving, except for a small region at one end of the sample. Figure 1: Schematic illustration of the experimental approach. Monochromatic light, emitted by a light-emitting diode, shines on a semitransparent mirror, which is used to split the beam allowing simultaneous measurements of the transmission through the sample and the intensity of the source. A diffusor is used to homogenize the illumination, before the entry window of the ultrahigh vacuum chamber. The transmitted light is registered by a CCD camera. The sample is covered with Al 2 O 3 to prevent hydrogen from entering and leaving, except for a small region at one end of the sample. Full size image The orientation of the vanadium single crystal with respect to the substrate [11] and the resulting diffusion direction is illustrated in Fig. 2 . The net diffusion direction of the hydrogen is in the [110] direction of the vanadium crystal, because of the directional relation of the crystallographic orientation to the catalytically active strip at one end of the sample. The total sample area is 10 mm×10 mm and the area of the catalytically active layer is ~3 mm×10 mm. The aspect ratio of the film thickness (50 nm) and the width of the stripe ensures equilibrated volume of hydrogen in the vanadium layer underneath the stripe that acts as a source or sink for the hydrogen diffusion. 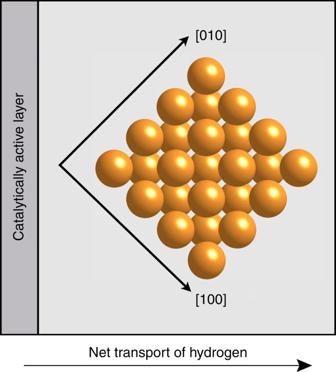Figure 2: Schematic top view of the sample and the orientation of the vanadium crystal. The epitaxial vanadium layer was grown on a MgO (001) substrate. The vanadium crystal is depicted by yellow spheres, and the in-plane lattice directions are indicated by arrows. The light grey area represents the oxide layer hindering the hydrogen uptake. The catalytically active stripe (dark grey) is parallel to one of the edges of the substrate, which results in a net diffusion of hydrogen in the [110] direction of the vanadium layer. Figure 2: Schematic top view of the sample and the orientation of the vanadium crystal. The epitaxial vanadium layer was grown on a MgO (001) substrate. The vanadium crystal is depicted by yellow spheres, and the in-plane lattice directions are indicated by arrows. The light grey area represents the oxide layer hindering the hydrogen uptake. The catalytically active stripe (dark grey) is parallel to one of the edges of the substrate, which results in a net diffusion of hydrogen in the [110] direction of the vanadium layer. Full size image Concentration profiles By recording the concentration profile at short-time intervals, we can follow their temporal evolution and in Fig. 3a we display the results obtained at 493 K. The horizontal axis represents the distance from the boundary where the hydrogen enters the sample, whereas the vertical axis specifies the time from the introduction of hydrogen in the chamber. The colour coding gives the concentration at any position and time during the measurements. The diffusion constant was determined from fitting the model described in equation (8) (see Methods section) to the data, using least squares minimization. The result is D =5(2)×10 −5 cm 2 s −1 using line fits and D =8(1)×10 −5 cm 2 s −1 using the whole dataset for c =0.045 H/V (atomic ratio). This value can be compared with chemical diffusion constants obtained from Gorsky experiments [12] that are 5.3(8)×10 −5 cm 2 s −1 for c =0.11 H/V and 9(2)×10 −5 cm 2 s −1 for c =0.02 H/V, respectively. In Fig. 3b, we display the calculated concentration as a function of position and time, using the results from the fitting. 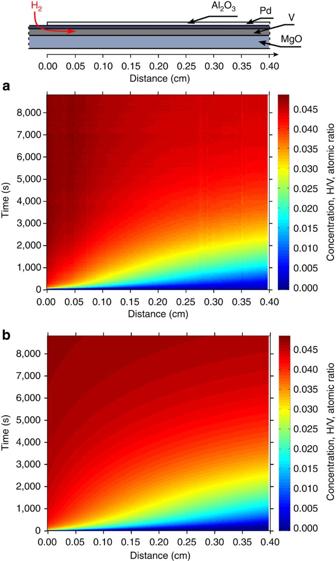Figure 3: Hydrogen concentration as a function of distance and time. The experimental results are shown in (a) and the solution to Fick's second law of diffusion in (b). The measurements were performed at 493 K and with an external hydrogen pressure of 0.4 mbar. The insert at the top illustrates the sample geometry, with the end of the Al2O3layer defining the starting point of the lateral diffusion. Figure 3: Hydrogen concentration as a function of distance and time. The experimental results are shown in ( a ) and the solution to Fick's second law of diffusion in ( b ). The measurements were performed at 493 K and with an external hydrogen pressure of 0.4 mbar. The insert at the top illustrates the sample geometry, with the end of the Al 2 O 3 layer defining the starting point of the lateral diffusion. Full size image The maximum equilibrium concentration in the sample is chosen by the temperature and the applied hydrogen pressure. This was used to perform diffusion measurements, at different temperatures, in the concentration range 0.01–0.50 H/V. Measurements of the lateral diffusion at concentrations of 0.5 H/V are shown in Supplementary Movie 1 . Given a film thickness of 50 nm or 330 monolayers of vanadium, a hydrogen concentration of 0.01 H/V corresponds to 3 effective monolayers of hydrogen. This sensitivity can be viewed as extraordinary and is unrivalled by any other measurement technique that we are aware of. We also notice large differences in the determined diffusion constants obtained at different hydrogen concentrations. To obtain a more quantitative comparison between the results and the fitting, we display the evolution of concentration as a function of both time and position in Fig. 4 . The evolution of the hydrogen concentration at different times is displayed in Fig. 4a , whereas the evolution at representative positions is illustrated in Fig. 4b . Besides the clearly identified lateral diffusion, a homogeneous increase in the concentration is clearly observed. This contribution was included in the simulations and amounts to about 1/20th of the total concentration. 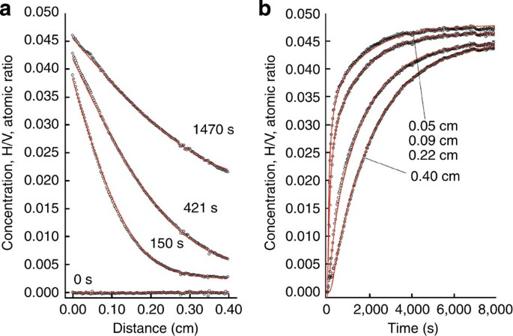Figure 4: Hydrogen concentration profiles at different times and positions. The concentration of hydrogen is plotted as the ratio of hydrogen to metal atoms over (a) distance and (b) time. Data is shown for different times and distances from the catalytic layer. The red lines represent least squares fits to the data using equation (8), as described in the Methods. Notice the sensitivity to the low amount of hydrogen with this method, where concentrations below 0.001 in H/V can easily be distinguished. Figure 4: Hydrogen concentration profiles at different times and positions. The concentration of hydrogen is plotted as the ratio of hydrogen to metal atoms over ( a ) distance and ( b ) time. Data is shown for different times and distances from the catalytic layer. The red lines represent least squares fits to the data using equation (8), as described in the Methods. Notice the sensitivity to the low amount of hydrogen with this method, where concentrations below 0.001 in H/V can easily be distinguished. Full size image The diffusion rates of hydrogen in metals are comparable to the mobility of liquid water molecules and many aspects of hydrogen in metals can be understood by viewing hydrogen as a lattice gas or as a lattice liquid [13] , [14] . Diffusion in randomly oriented crystals should yield a weighted average of the rates in the principal crystallographic directions, ignoring the effect of grain boundaries on the diffusion rate. Depending on the influence of the grain boundaries and other imperfections in the material, the obtained diffusion rates could be significantly affected. The origin of the observed homogeneous increase in the concentration has not been identified. Discontinuous coverage of the protecting oxide layer is a likely source, while we cannot exclude other possible contributions. The presence of two components does not affect the results of our analysis, as we can clearly separate the contribution from both channels. We also notice that, in the absence of the lateral information on the concentration, this separation would not be possible, which would affect the determined diffusion coefficients. Because of the discrete nature of the interstitial sites, the determined diffusion rate in different crystallographic directions will depend on the diffusion path in a single crystal. For example, in vanadium, the shortest distance between interstitial tetrahedral sites are the [110], [101] and [011] directions. These paths are the dominating directions of hydrogen transport in vanadium single crystals at low hydrogen concentrations. When calculating the relation between the diffusion- and the jump-rate, one needs to include these geometrical conditions. The results of the determined diffusion rates are therefore favourably compared with experiments using same boundary conditions. For example, a diffusion rate of 9(2)×10 −5 cm 2 s −1 for c =0.02 H/V was obtained with [110] as the dominating diffusion direction [12] , as compared with D =8(1)×10 −5 cm 2 s −1 for c =0.045 H/V obtained here. We notice an excellent agreement between the results from the two vastly different techniques. The approach described here opens up new possibilities to address new fundamental aspects of hydrogen diffusion, such as exploration of the directional and concentration dependence, the influence of strain, as well as imperfections on the chemical diffusion of hydrogen. Most transition metals exhibit a similar overall change in the electronic structure on hydrogen absorption (for example, ref. 15 ). It is therefore reasonable to conclude that this approach can be used for analysis of diffusion rates of hydrogen in a wide range of metals. The lower limit in thickness of the samples is in the monolayer range, whereas the upper limit is determined by the penetration depth of light. This approach is therefore highly suited for investigations of hydrogen in thin film structures. The use of this approach is not limited to determining the basic properties of hydrogen diffusion in materials. For example, metals with hydrogen as an added element often exhibit new and peculiar properties such as metal insulator transitions [5] , changes in magnetic properties [3] , [16] , [17] , changes in hardness and durability [18] , [19] , [20] , and modifications to superconducting properties [3] , [21] , to name a few. The possibility to determine the amount of hydrogen as a function of both position and time therefore opens up completely new avenues for combined measurements of concentration and different physical properties in thin films and multilayered structures. For example, the change in transmission can be used to determine the hydrogen concentration, whereas the rotation of polarization of the reflected beam can be used to determine the magnetization. In addition, the technique we describe opens up possibilities to investigate hydrogen migration as a function of strain, confinement and finite-size, all topics of importance for understanding the dynamics of hydrogen in confined spaces, such as nanomaterials. Diffusion equation A gradient in the chemical potential μ ( x,t ) (in one dimension) results in a current s ( x,t ) (ref. 22 ) where B ( c ) is the (concentration dependent) mobility and c is the concentration in atomic ratio H/V. Using the continuity relation (conservation of particles) Fick's second law is obtained as For a non-interacting lattice gas, where k B is the Boltzmann constant and T is the absolute temperature, the Einstein relation can be written as: [2] , [22] Because we are working with concentrations below 0.05 H/V and T =493 K far above any phase boundaries, we argue that the hydrogen behave essentially as non-interacting particles and this justifies dropping the c dependency of D and B . However, for experiments at higher concentrations, the so-called thermodynamic factor, f therm =( c / k B T )(∂ μ/ ∂ c ) has to be evaluated to determine the diffusivity. Finally, the common form of Fick's second law is obtained: The boundary and initial conditions for the sample geometry shown in Fig. 1 is where L is the distance from the end of the active area. These conditions imply the sample being free of hydrogen before the measurement starts, no hydrogen can flow through the end of the sample and a constant hydrogen supply is available at the other end of the sample, where the catalytically active palladium is facing the hydrogen gas. The solution of equation (6) with the boundary and initial conditions in equation (7) is given by refs 23 , 24 where erfc is the complementary error function. The solution depends only on three parameters, c 0 , L and D , the first two of which can be measured independently. Offsets in time and position were also added as fitting parameters to reduce the impact on artificial effects on the fits. The series converges fast and only k ≤10 need to be considered when comparing to the data. Representative solutions to the differential equation are shown in Fig. 4 along with experimental results. Film growth The 50 nm vanadium film was grown epitaxially on a double-sided polished MgO (001) 10 mm×10 mm×0.5 mm substrate using ultrahigh vacuum-based magnetron sputtering. The target purity was 99.98% and the base pressure in the system was 2×10 −7 Pa before deposition with the dominating residual gas being hydrogen. The sample was deposited from a vanadium target onto the substrate at 723 K on the heater. Argon, with purity better than 99.9999% at a pressure of 0.27 Pa was used as the sputtering gas. The sample was capped with a 5-nm palladium layer. The palladium was sputtered from a target with 99.99% purity after cooling the sample to room temperature. 10 nm amorphous Al 2 O 3 was subsequently deposited at 310 K with a piece of a microscope slide acting as a mask at one end of the sample. More detailed description of the growth and structural analysis can be found in ref. 11 . Concentration calibration The relation between hydrogen concentration and electronic structure is complex [25] , so we have resorted to a phenomenological approach of the conversion of optical transmission to hydrogen concentration, as described by Prinz et al . [9] : the optical transmission was determined at different hydrogen concentrations using an optical spectrometer. From these measurements, the optical response was established as a function of wavelength and concentration. A wavelength where the square root of pressure (Sievert's law) was proportional to the logarithm of the detected transmitted intensity was thereby identified ( λ =639 nm). Simultaneous measurements of the change in electrical resistivity were used to determine the change in concentration [26] . Verification of the concentration determination was obtained by comparing the results to previously determined isotherms, obtained from the hydrogen uptake in 50 nm thick vanadium films [9] , [26] , [27] . How to cite this article: Pálsson, G.K. et al . Using light transmission to watch hydrogen diffuse. Nat. Commun. 3:892 doi: 10.1038/ncomms1897 (2012).